Fabrication of enzyme-degradable and size-controlled protein nanowires using single particle nano-fabrication technique Protein nanowires exhibiting specific biological activities hold promise for interacting with living cells and controlling and predicting biological responses such as apoptosis, endocytosis and cell adhesion. Here we report the result of the interaction of a single high-energy charged particle with protein molecules, giving size-controlled protein nanowires with an ultra-high aspect ratio of over 1,000. Degradation of the human serum albumin nanowires was examined using trypsin. The biotinylated human serum albumin nanowires bound avidin, demonstrating the high affinity of the nanowires. Human serum albumin–avidin hybrid nanowires were also fabricated from a solid state mixture and exhibited good mechanical strength in phosphate-buffered saline. The biotinylated human serum albumin nanowires can be transformed into nanowires exhibiting a biological function such as avidin–biotinyl interactions and peroxidase activity. The present technique is a versatile platform for functionalizing the surface of any protein molecule with an extremely large surface area. Protein nanowires are drawing attention in various research fields, and several studies on drug delivery systems [1] , scaffolds for cell adhesion [2] and diagnosis [3] , [4] have been conducted using protein nanowires. Generally, self-assemblies of proteins and peptides have been employed to fabricate protein one-dimensional nanostructures because proteins and peptides are versatile building blocks for constructing well-defined one-dimensional nanostructures on the nano and submicrometer scale [5] . However, fabrication methods that take advantage of these self-assembly reactions cannot be applied to proteins and peptides which do not self-assemble. Furthermore, it is difficult to control the self-assembly reaction of protein molecules to provide nanowires of consistent length. Recently, it was reported that the size of a polymeric particulate antigen delivery system, a nanoparticle, was important for the efficient binding and uptake of particles by antigen-presenting cells, such as macrophages and dendritic cells [6] , [7] . Furthermore, the immune response changed both quantitatively and qualitatively depending on the particle size. Similarly, the specific interactions of protein nanowires with biological systems likely depend on the size of the protein nanowires. Thus, to fabricate protein nanowires that can act as a modulator, a fabrication method that gives uniformly sized nanowires is required. Living cells are surrounded by protein fibres, typically composed of collagen and fibronectin. These protein fibres regulate cellular responses through direct interactions with cell surface integrin receptors [8] , [9] . A recent study showed that the cellular response can be controlled by laying prepared fibronectin-based layer-by-layer nanometer-sized films directly on a cell surface; the degree of cellular response control depended on the thickness of the nanometer-sized films [10] . Thus, uniformly sized protein nanowires used as novel scaffolds should also be able to strictly control cellular responses. We have proposed a method for fabricating size-controlled nanowires by MeV-order high-energy charged particles; this methodology is referred to as the single particle nano-fabrication technique (SPNT) [11] , [12] , [13] , [14] . The MeV-order high-energy charged particles provide non-homogeneously deposited energy to irradiated materials along the particle trajectories, called ion tracks. In the past, the deposited energy in an ion track has been only applied to nuclear etching [15] , [16] or cancer radiotherapy [17] , [18] , in which the charged particles cause intense damage to the materials contacted. In contrast to these conservative applications of ion tracks, SPNT takes advantage of the deposited energy in an ion track to induce cross-linking reactions to fabricate nanowires. To date there have been no reports of the fabrication of nanowires composed of only proteins by ion beam irradiation because it was thought that charged particle radiation would destroy the fragile structures of proteins. The predicated cleavage of chemical bonds in protein molecules and the formation of new inter- and intra-molecular bonds would result in the loss of the biological activity of the proteins. SPNT is a method for fabricating one nanowire by a single charged particle whose energy can be controlled easily. It is, therefore, expected that adjusting the energy of the single charged particle will minimize damage to the structure of the protein and lead to retention of its biological activity. Here we report the fabrication and the characterization of enzyme-degradable and size-controlled protein nanowires by SPNT, and demonstrate their usabilities by conversion to the protein nanowires that show biological activity across large areas of the nanowire, taking advantage of the avidin–biotin interaction. Fabrication of HSA nanowires Human serum albumin (HSA) is the most abundant protein in human blood plasma and is a key protein involved in the biocompatibility of biomaterials. A single charged particle can fabricate one HSA nanowire along its trajectory. Non-cross-linked HSA can be removed with phosphate-buffered saline (PBS) ( Fig. 1a ). After drying, the surface of the irradiated film was observed by atomic force microscopy (AFM). The AFM images suggested that HSA nanowires with a cross-linked structure were fabricated by the ion beam ( Fig. 1b ). The density of the HSA nanowires increased with increasing fluence of the charged particle ( Fig. 1b–e ); thus, by adjusting the fluence of the charged particle, the density of the HSA nanowires can be easily controlled. The irradiated HSA film showed a broad electron spin resonance (ESR) signal, as shown in Fig. 1f , indicating the presence of a radical generated by the irradiation. The g -value of this radical was 2.0058, and the spectrum was similar to that of the γ-irradiated egg albumin radical [19] . This results suggest that the radical species derived from HSA is involved in the inter- and/or intra-molecular cross-linking reaction. The structural analysis of the HSA molecules in the nanowires was carried out by using a circular dichroism (CD) spectroscopy and Fourier transform infrared–attenuated total reflectance (FTIR–ATR) spectroscopy. It is likely that the HSA molecules in the nanowires maintain the secondary strcture [20] ( Supplementary Fig. 1 ). 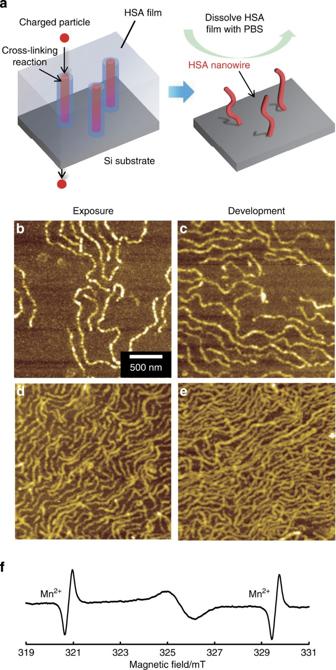Figure 1: Formation of HSA nanowires. (a) Process for fabricating HSA nanowires by SPNT. AFM images of the HSA nanowires formed by irradiation of a HSA spin-coated film with a 320 MeV102Ru18+-ion beam at a fluence of (b) 1.0 × 108, (c) 3.0 × 108, (d) 7.0 × 108and (e) 1.0 × 109ions cm−2. (f) ESR spectrum of HSA drop-cast film irradiated with an ion beam at a fluence of 5.0 × 109ions cm−2. Figure 1: Formation of HSA nanowires. ( a ) Process for fabricating HSA nanowires by SPNT. AFM images of the HSA nanowires formed by irradiation of a HSA spin-coated film with a 320 MeV 102 Ru 18+ -ion beam at a fluence of ( b ) 1.0 × 10 8 , ( c ) 3.0 × 10 8 , ( d ) 7.0 × 10 8 and ( e ) 1.0 × 10 9 ions cm −2 . ( f ) ESR spectrum of HSA drop-cast film irradiated with an ion beam at a fluence of 5.0 × 10 9 ions cm −2 . Full size image The effect of the nature and energy of the charged particle on the fabrication of HSA nanowires was examined by varying the ion beam. 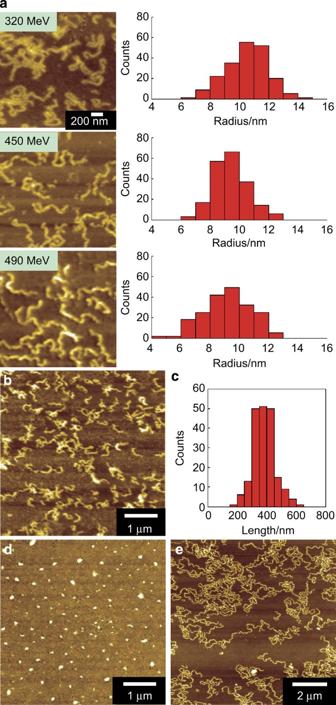Figure 2: Effects of the type of charged particle and the film thickness. (a) AFM images and radius distributions of HSA nanowires formed by irradiation of an HSA spin-coated film with various ion beams. The irradiation ion beams were 320 MeV102Ru18+, 450 MeV129Xe23+and 490 MeV192Os30+. (b) AFM image and (c) length distribution of the HSA nanowires formed by irradiation of a 500-nm-thick HSA spin-coated film with a 490 MeV192Os30+-ion beam at a fluence of 1.0 × 109ions cm−2. AFM images of (d) HSA nanodots and (e) high aspect ratio HSA nanowires. Figure 2a shows AFM images of HSA nanowires formed by irradiation of an HSA spin-coated film with various ion beams. The average radius of the nanowires was 10.5±1.4, 9.4±1.2 and 9.1±1.6 nm following radiation with a 320 MeV 102 Ru 18+ , 450 MeV 129 Xe 23+ and 490 MeV 192 Os 30+ ion beam, respectively. The following equation has been proposed for estimating the diameter (2 r ) of HSA nanowires produced by cross-linking reactions induced by a high-energy single particle releasing its energy along the trajectory; note that LET (linear energy transfer), (eV nm −1 ) is the average energy deposition of linear energy transfer [14] : Figure 2: Effects of the type of charged particle and the film thickness. ( a ) AFM images and radius distributions of HSA nanowires formed by irradiation of an HSA spin-coated film with various ion beams. The irradiation ion beams were 320 MeV 102 Ru 18+ , 450 MeV 129 Xe 23+ and 490 MeV 192 Os 30+ . ( b ) AFM image and ( c ) length distribution of the HSA nanowires formed by irradiation of a 500-nm-thick HSA spin-coated film with a 490 MeV 192 Os 30+ -ion beam at a fluence of 1.0 × 10 9 ions cm −2 . AFM images of ( d ) HSA nanodots and ( e ) high aspect ratio HSA nanowires. Full size image where A is Avogadro’s number, e is Napier’s constant, Mw is the molecular weight of HSA, ρ (g nm −3 ) is the density of the HSA film, G ( x ) (100 eV) −1 is the number of cross-links induced by a radiation-deposited energy of 100 eV, and r c and r p are the radii of the core and penumbra areas, defined from the equipartition theorem of collisions of charged particles with matter. The estimate of the diameter of the nanowire derived from equation (1) depends only on the value of LET of the incident particle. The values of LET are calculated as 7,500, 9,300 and 12,300 eV nm −1 for 320 MeV 102 Ru 18+ , 450 MeV 129 Xe 23+ and 490 MeV 192 Os 30+ , respectively, in the HSA film by SRIM 2010 simulation code. The cross-linking efficiency of G ( x ) is also derived from equation (1) from observed values of r , estimated as G ( x )=1.5, 1.3 and 1.3 (100 eV) −1 for the film with a 320 MeV 102 Ru 18+ , 450 MeV 129 Xe 23+ and 490 MeV 192 Os 30+ ion beam, respectively. There was a little change in G ( x ) between the ion beams, and the HSA nanowires can be stably fabricated regardless of the type of ion beam used. Moreover, the HSA nanowires maintain the shapes over 3 months in ambient conditions and over 12 h in PBS ( Supplementary Fig. 2 ). The results show that HSA is a suitable biomaterial for the generation of protein nanowires. To examine the homogeneity of the HSA nanowires, their lengths were estimated from an AFM image ( Fig. 2b ). There was little variability in the length among the HSA nanowires; their average length was 380±70 nm, which was slightly shorter than the film thickness (500 nm), suggesting small shrinkage effects in the nanowires caused by the cross-linking reactions and the development procedures ( Fig. 2c ). The ratio of shrinkage (0.82) was identical to that of nanowires with extremely high aspect ratio ( Supplementary Fig. 3 ). Thus, using SPNT, the length of the nanowires generated is in direct proportion to the film thickness: by adjusting the thickness of the film, nanowires of various lengths can be fabricated, from HSA nanodots to HSA nanowires with extremely high aspect ratios of over 1,000 ( Fig. 2d,e ). In contrast, it is difficult to fabricate homogeneous protein nanowires of controlled length over a large area by the self-assembly of proteins and peptides. Thus, the SPNT method is expected to provide protein nanowires that can be used to investigate biological responses [1] , [2] and have possibility to fabricate novel drug carrier and scaffolds. Degradation of HSA nanowires with trypsin Susceptibility to degradation is a very important factor for biomaterials. Trypsin is a pancreatic serine protease that hydrolyses the peptide bond on the carboxyl side of positively charged lysine and arginine residues in peptides and proteins [21] . The HSA nanowires fabricated by SPNT are enzymatically degradable. To evaluate the enzymatic susceptibility of HSA nanowires, the HSA nanowires were incubated with trypsin and their surface was observed by AFM ( Fig. 3a ). The HSA nanowires lost their original shapes within 10 min, and no nanowires were evident following incubation for 30 min. This result indicated clearly that HSA nanowires are degraded by trypsin ( Fig. 3b ). 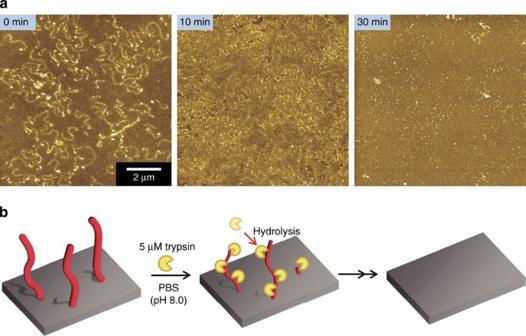Figure 3: Degradation of HSA nanowires with trypsin. (a) AFM images of hydrolysates of HSA nanowires after immersion in 5 μM trypsin solution at 37 °C for 0, 10 and 30 min (left to right). (b) Schematic depiction of the degradation of HSA nanowires by trypsin. Figure 3: Degradation of HSA nanowires with trypsin. ( a ) AFM images of hydrolysates of HSA nanowires after immersion in 5 μM trypsin solution at 37 °C for 0, 10 and 30 min (left to right). ( b ) Schematic depiction of the degradation of HSA nanowires by trypsin. Full size image Preparation of biotinylated HSA nanowires The avidin–biotin interaction is well known for its extraordinary affinity ( K a=10 15 M −1 ) [22] , [23] . We modified the surface of the HSA nanowires by introducing the biotinyl group so that the nanowires could specifically interact with avidin ( Fig. 4a ). The average radius of the HSA nanowires, the biotinylated HSA nanowires and the biotinylated HSA nanowires incubated with avidin were 8.4±1.7, 9.0±2.0 and 12.0±2.4 nm, respectively ( Fig. 4b–d ). The increase in diameter (6.0 nm) of the biotinylated HSA nanowires corresponds to the size of avidin (5.6 × 5.0 × 4.0 nm) [24] , indicating that avidin was bound to the biotinylated HSA nanowires. Furthermore, avidin has four biotin-binding sites. There would thus be a tendency for biotinylated HSA nanowires bound to avidin to aggregate. 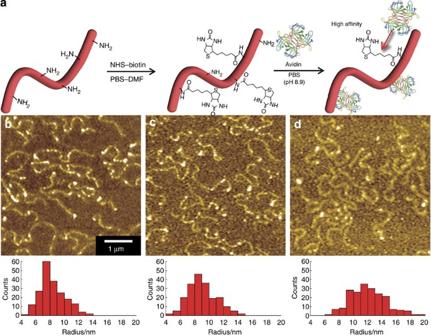Figure 4: Fabrication of biotinylated HSA nanowires. (a) Scheme showing the surface modification of HSA nanowires by introducing biotinyl groups and the affinity between biotinylated HSA nanowires and avidin. AFM images and radius distributions of (b) HSA nanowires, (c) biotinylated HSA nanowires and (d) biotinylated HSA nanowires after immersion in an avidin solution at room temperature for 30 min. Figure 4: Fabrication of biotinylated HSA nanowires. ( a ) Scheme showing the surface modification of HSA nanowires by introducing biotinyl groups and the affinity between biotinylated HSA nanowires and avidin. AFM images and radius distributions of ( b ) HSA nanowires, ( c ) biotinylated HSA nanowires and ( d ) biotinylated HSA nanowires after immersion in an avidin solution at room temperature for 30 min. Full size image SPNT as a versatile tool for protein nanowires SPNT was applied to three proteins: bovine serum albumin (BSA), ovalbumin (OVA) and avidin films. BSA and OVA films provided clearly observable BSA and OVA nanowires, similar to HSA nanowires ( Fig. 5a,b ). On the other hand, only a few nanowires were observed using avidin ( Fig. 5c ). It is likely that the avidin nanowires broke because of low mechanical strength and were removed during the development process. These results suggest that the formation of nanowires by SPNT is protein-dependent. 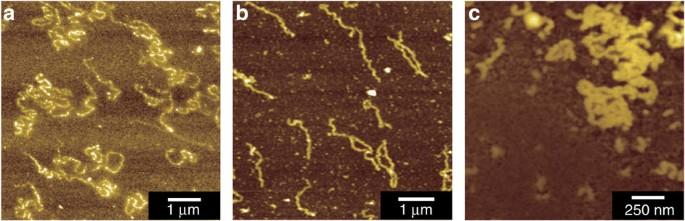Figure 5: Fabrication of various protein nanowires. AFM images of protein nanowires based on (a) BSA, (b) OVA, (c) avidin. Figure 5: Fabrication of various protein nanowires. AFM images of protein nanowires based on ( a ) BSA, ( b ) OVA, ( c ) avidin. Full size image Interaction between HSA–avidin nanowires and biotin We attempted to improve the mechanical strength of the avidin nanowires by mixing avidin and HSA. 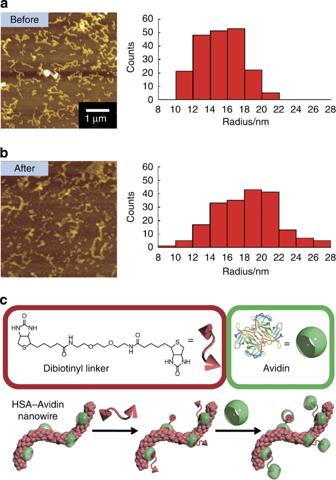Figure 6: Interaction between an HSA–avidin nanowire and biotin. AFM images and radius distributions of HSA–avidin (HSA:avidin=1:1) (a) before and (b) after immersion into a dibiotinyl linker solution, followed by immersion into an avidin solution. This process was repeated three times. (c) Scheme showing the surface modification of HSA–avidin nanowires using a dibiotinyl linker and avidin. Figure 6a shows an AFM image of HSA–avidin nanowires obtained using a 1:1 mixture of HSA and avidin. The results demonstrate that nanowires of an appropriate mechanical strength can be fabricated by mixing HSA with other proteins. To examine whether HSA–avidin nanowires exhibit specific interactions with biotin, the radius of the nanowires was measured after immersing them three times into dibiotynyl linker and avidin solution. The average radius of HSA–avidin nanowires increased from 15.2±2.4 to 18.3±3.5 nm following this treatment ( Fig. 6a,b ), clearly indicating that HSA–avidin nanowires exhibit specific interactions with biotin ( Fig. 6c ). Avidin was thus immobilized through chemical linkages formed by ion beam irradiation, but its biotin-binding site was not destroyed. Figure 6: Interaction between an HSA–avidin nanowire and biotin. AFM images and radius distributions of HSA–avidin (HSA:avidin=1:1) ( a ) before and ( b ) after immersion into a dibiotinyl linker solution, followed by immersion into an avidin solution. This process was repeated three times. ( c ) Scheme showing the surface modification of HSA–avidin nanowires using a dibiotinyl linker and avidin. Full size image Functionalization of biotinylated HSA nanowires The biotinylated HSA nanowires can be converted to various types of functionalized nanowires by taking advantage of the strong interaction between biotin and streptavidin and avidin. These nanowires can bind fluorescent probes, and exhibit biological activities due to their binding of functional proteins such as enzymes, binding proteins and antibodies. For example, biotinylated HSA nanowires were incubated with streptavidin conjugated with Alexa Fluor 488 (fluorescent probe); after washing to remove unbound reagent, fluorescent nanowires were obtained ( Fig. 7a ). The emission spectrum of the nanowires was identical to that of the unbound fluorescent probe ( Fig. 7b ). A second example of the functionalization of protein nanowires was demonstrated using horseradish peroxidase (HRP), which is widely used in bioanalytical analyses due to its high substrate turnover, which provides signal amplification [25] , [26] . Biotinylated HSA nanowires were treated in a manner similar to that described above with HRP conjugated with streptavidin (HRP–streptavidin) to give nanowires with peroxidase activity ( Fig. 7a ). HSA nanowires without biotin were also treated with HRP–streptavidin. The enzymatic activity of biotinylated HSA nanowires treated with HRP–streptavidin was 10 times larger than that of HSA nanowires treated with HRP–streptavidin ( Fig. 7c ). This is due to the HRP of the HRP–streptavidin complex being bound to the biotinylated nanowire through the strong interaction between the biotin moiety and the streptavidin moiety. The weak enzymatic activity of the HSA nanowires treated with HRP–streptavidin can be attributed to nonspecific binding of HRP–streptavidin to the large surface area of the HSA nanowire [3] . 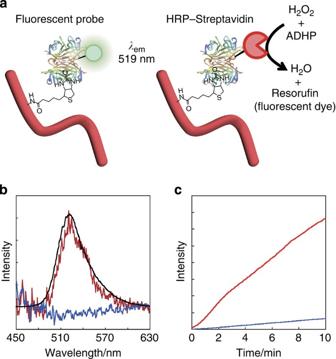Figure 7: Biotinylated HSA nanowires conjugated with fluorescence probes or enzymes. (a) Scheme showing binding of Alexa Fluor 488-conjugated streptavidin (Fluorescent probe) and streptavidin-conjugated HRP (HRP–streptavidin) onto biotinylated HSA nanowires. (b) Emission spectra of fluorescent probe (excitation at 355 nm). (Red) biotinylated HSA nanowires+fluorescent probe; (blue) HSA nanowires+fluorescent probe; (black) fluorescent probe. (c) Time course of the enzymatic reaction. (Red) biotinylated HSA nanowires+HRP–streptavidin; (blue) HSA nanowires+HRP–streptavidin. The enzymatic reaction was monitored by measuring the fluorescence at 585 nm (excitation at 570 nm). Figure 7: Biotinylated HSA nanowires conjugated with fluorescence probes or enzymes. ( a ) Scheme showing binding of Alexa Fluor 488-conjugated streptavidin (Fluorescent probe) and streptavidin-conjugated HRP (HRP–streptavidin) onto biotinylated HSA nanowires. ( b ) Emission spectra of fluorescent probe (excitation at 355 nm). (Red) biotinylated HSA nanowires+fluorescent probe; (blue) HSA nanowires+fluorescent probe; (black) fluorescent probe. ( c ) Time course of the enzymatic reaction. (Red) biotinylated HSA nanowires+HRP–streptavidin; (blue) HSA nanowires+HRP–streptavidin. The enzymatic reaction was monitored by measuring the fluorescence at 585 nm (excitation at 570 nm). Full size image Size-controlled protein nanowires were fabricated by ion beam irradiation of an HSA film. A broad ESR signal of the irradiated HSA film indicates the presence of a radical generated by the irradiation. The clear ESR spectrum observed even at room temperature [19] shows intermolecular cross-linking promoted by radical coupling reactions. The structural analysis by CD spectroscopy and FTIR–ATR spectroscopy suggest that the HSA molecules incorporated into the nanowires maintain the secondary structure [20] . The HSA nanowires can be stably fabricated regardless of the type of ion beam used. Since the HSA nanowires could be degraded by trypsin, HSA is a suitable biomaterial for the generation of protein nanowires. Clearly observable BSA nanowires and OVA nanowires were fabricated similarly. On the other hand, only a few nanowires were observed using avidin, suggesting that the formation of nanowires by SPNT is protein-dependent. Biotinylated HSA nanowires were prepared by introducing the biotinyl group into the HSA nanowires, and the biotinylated HSA nanowires bound avidin. The HSA–avidin nanowires of appropriate mechanical strength can be fabricated by mixing HSA with avidin. Avidin was immobilized in the HSA–avidin nanowires through chemical linkages formed by ion beam irradiation. The biotin-binding site of the avidin moieties was not destroyed and retained the ability to bind specifically with biotin, despite irradiation with MeV-order high-energy charged particles. To the best of our knowledge, this is the first report of fabrication of protein nanowires retaining their bio-activity following heavy ion irradiation of the protein. The biotinylated HSA nanowires could be converted to fluorescent nanowires and to nanowires with peroxidase activity [25] , [26] by treating the wires with a fluorescent probe or with HRP–streptavidin, respectively. The conjugation of proteins with biotin or streptavidin is an established technique [22] , [23] , and many biotinylated proteins and streptavidin-conjugated proteins are commercially available. Since the HSA–avidin nanowires and the biotinylated HSA nanowires can be transformed very easily into nanowires with various biological functions, these may also be of commercial interest. SPNT is thus expected to be very effective for the fabrication of protein nanowires exhibiting various biological functions for creating diverse biomaterials. Furthermore, nanowires composed of protein and synthetic polymer can also be fabricated by SPNT ( Supplementary Fig. 4 ). Accordingly, SPNT is expected to provide homogeneous multi-functional nanowires which are otherwise difficult to fabricate, by combining a functional polymer with protein. These nanowires will contribute to tremendous improvement in the sensitivity of enzyme-linked immunoassay because of their large surface areas. Furthermore, they can be used for highly sensitive clinical diagnosis of diseases which include multiple and quantitative enzymes immobilization, such as inflammation system and blood coagulation system. Reagents HSA, BSA, and OVA from egg were purchased from Sigma-Aldrich. Avidin from chicken egg white was purchased from Calzyme Laboratories. Trypsin from porcine pancreas was purchased from Nacalai Tesque. Biotin N -hydroxysuccinimide ester (NHS-biotin), HRP conjugated with streptavidin (HRP–streptavidin) and QuantaRed Enhanced Chemifluorescent HRP Substrate kit were purchased from Thermo Fisher Scientific. Streptavidin conjugated with Alexa Fluor 488 was purchased from Life Technologies. D -Biotin was purchased from AnaSpec. 3,6-Dioxaoctane-1,8- N -dibiotinamide (dibiotinyl linker) was prepared using literature methods from D -biotin [27] . All other reagents and solvents were purchased from Wako Pure Chemical. Fabrication of the protein nanowires on a Si substrate Protein films on a silicon (Si) wafer (0.5 × 0.5 cm 2 ) were prepared by spin-casting with HSA, BSA, OVA, or avidin or a mixture of HSA and avidin (HSA:avidin=1:1), in water. The thickness of the films was confirmed using a Dektak 150 Stylus Surface Profiler (ULVAC, Japan). The films on a Si wafer were irradiated in a vacuum chamber (<10 −4 Pa) with 320 MeV 102 Ru 18+ , 450 MeV 129 Xe 23+ or 490 MeV 192 Os 30+ ion beams from the cyclotron accelerator at Takasaki Advanced Radiation Research Institute, Japan Atomic Research Agency. The fluence of the incident ions varied from 1.0 × 10 8 to 1.0 × 10 9 ions cm −2 . After irradiation, the samples were developed using PBS, pH 7.4 for between 3 and 30 min and dried at room temperature. For the fabrication of HSA nanowires with extremely high aspect ratios of over 1,000, an HSA drop-cast film on a Si wafer was irradiated in a vacuum chamber with a 490 MeV 192 Os 30+ ion beam at a fluence of 1.0 × 10 8 ions cm −2 . After irradiation, the samples were developed using PBS (pH 7.4) for 6 h and dried at room temperature. AFM observation of protein nanowires The protein nanowires on a Si substrate were observed by AFM. The AFM images were obtained with a SPI-4000 operated in tapping mode in air at room temperature. The radius of the cross-section ( r ) for any given nanowire was estimated from the following equation: where r 1 and r 2 are the half width and half height at half maximum of the AFM trace of the cross-section, respectively. The lengths of the protein nanowires on a Si substrate were estimated using the following protocol: (1) set an inscribed circle onto each AFM tone of a nanowire in an AFM image, (2) evaluate the radii of gyration ( S ) for at least 100 nanowires and (3) derive the total length of the nanowires ( L ) from the two-dimensional worm-like chain model and average over the nanowires, thus obtaining the average length (ln< L 2 >= b ln (6< S 2 >)). The excluded volume effects of the nanowires were disregarded in the evaluation processes; this simplification was supported by the presence of partially self-overlapping images of nanowires on the substrate. The scaling parameter b was estimated from an AFM trace of short nanowires (<100 nm) using an applicable stiff rod-like model for the analysis. ESR measurements of an HSA film irradiated with an ion beam For the ESR measurements, an HSA drop-cast film irradiated with a 490 MeV 192 Os 30+ -ion beam at a fluence of 5.0 × 10 9 ions cm −2 was placed in a quartz-glass sample tube. The ESR spectra were obtained with a JEOL JES-FA200 ESR spectrometer coupled with a computer for data acquisition and instrument control. The signal intensity was corrected using a Mn 2+ marker. Structural analysis of HSA nanowires CD spectra of HSA nanowires suspended in PBS (pH 7.4) was recorded with a JASCO J-820AC spectropolarimeter at 25 °C. Twenty four scans were accumulated at a scan speed of 20 nm min −1 . As for 10 μM HSA in PBS, two scans were accumulated at a scan speed of 50 nm min −1 . FTIR–ATR of HSA nanowires on Si substrate was recorded with a NEXUS 470 FTIR spectrometer. The interferograms were coded 512 times and Fourier-transformed at a resolution of 4 cm −1 . For HSA, the interferograms were coded 32 times. Degradation of HSA nanowires with trypsin HSA nanowires on a Si wafer were formed by ion beam irradiation of the HSA spin-coated film at a fluence of 3.0 × 10 8 ions cm −2 . The HSA nanowires were incubated with 5 μM trypsin in PBS (pH 8.0) at 37 °C for 10 or 30 min and washed with water. After drying at room temperature, the hydrolysates of the HSA nanowires on the Si substrate were observed by AFM. Preparation of biotinylated HSA nanowires The HSA nanowires were fabricated on a Si substrate as described above. The substrates were then immersed in a mixture of PBS (pH 7.4) and N,N -dimethylformamide solution of NHS-biotin (10 mM) (PBS: N,N -dimethylformamide=1:1) for 2 h at room temperature, then carefully washed with water. The biotinylated HSA nanowires on the Si substrate were immersed in 10 μM avidin solution in PBS (pH 8.9) for 30 min, then washed with water. After drying at room temperature, the radii of the nanowires were evaluated by AFM. Interaction between HSA–avidin nanowires and biotin HSA–avidin nanowires were prepared by ion beam irradiation of a spin-coated film of a mixture of HSA and avidin (HSA:avidin=1:1) as described above. The HSA–avidin nanowires were immersed in 10 μM dibiotinyl linker in a mixture of PBS (pH 7.4) and dimethyl sulfoxide (PBS:dimethyl sulfoxide=1:1) for 30 min and carefully washed with water. The nanowires treated with dibiotinyl linker were immersed in 10 μM avidin in PBS for 30 min. The procedure was repeated three times. After each immersion, the substrate was carefully washed with water. The radii of the nanowires were evaluated by AFM. Preparation of biotinylated HSA nanowires with fluorescence The biotinylated HSA nanowires on a Si substrate (1.5 × 0.7 cm 2 ) were incubated with 50 μg cm −3 Alexa Fluor 488-conjugated streptavidin in 0.1 M potassium phosphate buffer (pH 7.0) at 25 °C for 30 min. After washing with the same buffer three times, the emission spectrum of the nanowires was measured. The excitation wavelength was 355 nm. Preparation of biotinylated HSA nanowires with HRP The biotinylated HSA nanowires on a Si substrate (1.5 × 0.7 cm 2 ) were incubated with 100 ng cm −3 HRP–streptavidin in 10 mM potassium phosphate buffer containing 0.15 M sodium chloride (pH 7.0) at 25 °C for 30 min, then the nanowires were washed with the same buffer three times. A QuantaRed Enhanced Chemifluorescent HRP Substrate kit (Thermo Scientific) was used for assaying the HRP activity [26] . The nanowires was dipped into a mixture of 1.8 cm 3 of 0.1 M potassium phosphate buffer (pH 7.0) and 0.2 cm 3 of substrate solution containing 10-acetyl 3,7-dihydroxyphenoxazine and hydrogen peroxide. The enzymatic reaction mixture was stirred at 800 r.p.m. The time course of the enzymatic reaction was monitored continuously by measuring the fluorescence at 585 nm (excitation at 570 nm). How to cite this article: Omichi, M. et al. Fabrication of enzyme-degradable and size-controlled protein nanowires using single particle nano-fabrication technique. Nat. Commun. 5:3718 doi: 10.1038/ncomms4718 (2014).